Hypoxia-mediated downregulation of miRNA biogenesis promotes tumour progression Cancer-related deregulation of miRNA biogenesis has been suggested, but the underlying mechanisms remain elusive. Here we report a previously unrecognized effect of hypoxia in the downregulation of Drosha and Dicer in cancer cells that leads to dysregulation of miRNA biogenesis and increased tumour progression. We show that hypoxia-mediated downregulation of Drosha is dependent on ETS1/ELK1 transcription factors. Moreover, mature miRNA array and deep sequencing studies reveal altered miRNA maturation in cells under hypoxic conditions. At a functional level, this phenomenon results in increased cancer progression in vitro and in vivo , and data from patient samples are suggestive of miRNA biogenesis downregulation in hypoxic tumours. Rescue of Drosha by siRNAs targeting ETS1/ELK1 in vivo results in significant tumour regression. These findings provide a new link in the mechanistic understanding of global miRNA downregulation in the tumour microenvironment. MicroRNAs (miRNAs) are evolutionarily conserved small RNA molecules intricately involved in gene regulation [1] , [2] . Considering the broad functional involvement of miRNAs in cellular homeostasis, it is not surprising that cancer cells have altered miRNA levels [2] , [3] and that miRNAs are extensively involved in cancer progression [4] , [5] . Although global miRNA downregulation in cancer has been reported [2] , [6] , [7] , the mechanism of this downregulation is not fully understood. Drosha and Dicer are key enzymes involved in miRNA biogenesis. We and others have previously shown that downregulation of Drosha and Dicer in ovarian, lung and breast cancer is associated with poor patient outcome [7] , [8] , [9] , [10] , [11] . Although individual regulators of Dicer (for example, let7) [12] , [13] , [14] , [15] , [16] have been implicated, the underlying mechanisms are poorly defined. In this study, we identify new mechanisms of deregulation of miRNA biogenesis, whereby hypoxia results in reduced Drosha and Dicer. Specifically, we found that Drosha downregulation under hypoxic conditions is mediated by ETS1/ELK1 and promoter methylation. Moreover, Dicer is downregulated by epigenetic mechanisms as defined by van den Beucken et al. [17] This study uncovers precise mechanisms by which intra-tumoral hypoxia suppresses miRNA expression by disrupting the miRNA biogenesis machinery. Hypoxia downregulates miRNA biogenesis First, we determined whether tumours have stable heterogeneity with regard to Drosha and Dicer. We examined single-cell clones of A2780 ovarian cancer cells and found heterogeneous expression of Drosha and Dicer ( Supplementary Fig. 1a ). To understand the functional implications of this heterogeneity, we expanded and injected two single-cell clones of A2780 cells into the peritoneal cavity of mice (Clones 2 and 4). On analysis of individual tumour samples, we observed that each sample had varying Drosha and Dicer expression levels compared with the expression of clones at the time of injection ( Supplementary Fig. 1b ). This prompted us to consider whether changes in expression levels of Drosha and Dicer could be dynamic and potentially affected by the tumour microenvironment. Considering the critical role of hypoxia in the tumour microenvironment [18] , [19] , [20] , we tested levels of hypoxia in the clones with low Drosha and Dicer, also A2780 tumour samples using the hypoxia marker carbonic anhydrase 9 (CA9). In the cell clones, in vitro , we observed variable levels of CA9 with small magnitude of changes ( Supplementary Fig. 1c ). In contrast, the tumour samples with low Drosha and Dicer levels displayed significantly increased expression of CA9, which was inversely correlated with Drosha ( Supplementary Fig. 1d ) and Dicer ( Supplementary Fig. 1e ) levels. We next tested the effect of hypoxia on Drosha and Dicer levels using various cancer cell lines. In multiple cell lines exposed to hypoxia, we observed marked reductions in Drosha and Dicer messenger RNA and protein levels ( Fig. 1a,b and Supplementary Fig. 2a–e ). This observed downregulation was consistent across several time points ( Supplementary Fig. 2e ); the 48-h time point was selected for all subsequent experiments. Drosha and Dicer levels were significantly increased after cells were restored to normoxic conditions, demonstrating the dynamic nature of the downregulation ( Supplementary Fig. 2f ). To test the possibility of hypoxia-inducible factor-α (HIF1α) dependency in Drosha and Dicer downregulation, we examined Drosha and Dicer expression levels in mouse embryonic fibroblasts with wild-type HIF1α or HIF1α-knockout cultured under normoxic or hypoxic conditions. HIF1α-knockout mouse embryonic fibroblasts showed complete abrogation in Drosha downregulation under hypoxia exposure and partial abrogation in Dicer downregulation ( Supplementary Fig. 3a ), suggesting that Drosha downregulation is highly dependent on HIF1α. In addition, siHIF1α significantly rescued Drosha levels in hypoxia-exposed A2780 cells and Dicer levels were partially rescued ( Supplementary Fig. 3b ). These data were further supported by stabilization of HIFα by CoCl 2 in A2780 cells under normoxia. Increased CA9 was observed, followed by Drosha and Dicer downregulation in CoCl 2 -treated samples compared with control cells ( Supplementary Fig. 3c ). These data suggest a HIF1α-dependent downregulation of Drosha. We observed Dicer is downregulated in CoCl 2 -treated cells, but the mechanisms for this effect are largely independent of HIF1α stabilization, as reported by van den Beucken et al. 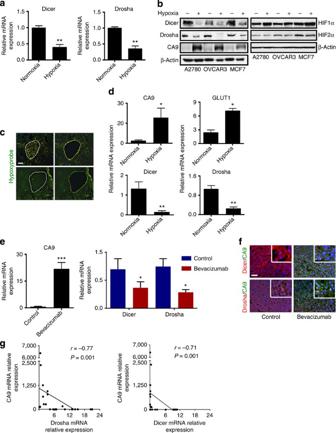Figure 1: Hypoxia downregulates Drosha and Dicerin vitroandin vivo. (a) Drosha and Dicer mRNA expression levels under hypoxic conditions (1% oxygen, 48 h) in A2780 cells. (b) Protein expression of Dicer, Drosha, hypoxia marker CA9, HIF1α and HIF2α under hypoxic conditions in A2780, OVCAR3 and MCF7 cells. (c) Laser microdissection of hypoxic areas of tumours, guided by Hypoxyprobe staining (green). Scale bar, 500 μm. (d) mRNA expression levels of hypoxia markers CA9 and GLUT1, as well as Dicer and Drosha expression levels, in normoxic and hypoxic regions of tumours isolated using microdissection. (e) mRNA expression levels of CA9, Drosha and Dicer in A2780 mouse tumours treated with bevacizumab. (f) Protein expression levels of Dicer (red), Drosha (red) and CA9 (green) in A2780 mouse tumour samples treated with bevacizumab compared with untreated controls. Nucleus indicated in blue. Scale bar, 200 μm. (g) Pearson correlation between Dicer and Drosha mRNA expression levels and hypoxia marker CA9 levels (n=30). All images shown are representative and data are presented as mean±s.e.m. ofn≥3 experimental groups. *P<0.05, **P<0.01, ***P<0.001 (Studentt-test). [17] Figure 1: Hypoxia downregulates Drosha and Dicer in vitro and in vivo . ( a ) Drosha and Dicer mRNA expression levels under hypoxic conditions (1% oxygen, 48 h) in A2780 cells. ( b ) Protein expression of Dicer, Drosha, hypoxia marker CA9, HIF1α and HIF2α under hypoxic conditions in A2780, OVCAR3 and MCF7 cells. ( c ) Laser microdissection of hypoxic areas of tumours, guided by Hypoxyprobe staining (green). Scale bar, 500 μm. ( d ) mRNA expression levels of hypoxia markers CA9 and GLUT1, as well as Dicer and Drosha expression levels, in normoxic and hypoxic regions of tumours isolated using microdissection. ( e ) mRNA expression levels of CA9, Drosha and Dicer in A2780 mouse tumours treated with bevacizumab. ( f ) Protein expression levels of Dicer (red), Drosha (red) and CA9 (green) in A2780 mouse tumour samples treated with bevacizumab compared with untreated controls. Nucleus indicated in blue. Scale bar, 200 μm. ( g ) Pearson correlation between Dicer and Drosha mRNA expression levels and hypoxia marker CA9 levels ( n =30). All images shown are representative and data are presented as mean±s.e.m. of n ≥3 experimental groups. * P <0.05, ** P <0.01, *** P <0.001 (Student t -test). Full size image In RNA samples isolated from microdissected hypoxic regions of A2780 tumour samples, we observed significantly increased expression of hypoxia markers, CA9 and GLUT1. In the same RNA samples, we observed 60% downregulation of Drosha and Dicer ( Fig. 1c,d ). These data support our finding that hypoxia is an important regulator of Drosha and Dicer downregulation in cancer. As previous studies have shown that anti-vascular endothelial growth factor (VEGF) therapies can increase hypoxia [21] , we assessed Drosha and Dicer levels in mouse tumour samples following treatment with bevacizumab. We observed increased CA9 expression and, consequently, significantly decreased Drosha and Dicer expression levels in tumours treated with bevacizumab compared with untreated controls ( Fig. 1e,f ). To determine whether similar findings extend to clinical samples, we analysed expression levels of Drosha, Dicer and a hypoxia marker CA9 in human tumour samples ( N =30). Results showed a significant inverse correlation between CA9 and Drosha and Dicer levels ( Fig. 1g ). Effect of hypoxia on miRNA levels and clinical outcomes We next considered whether Drosha or Dicer downregulation leads to impaired miRNA biogenesis by carrying out miRNA microarray analysis of samples exposed to hypoxia or normoxia. On analysis of mature miRNA array data, we observed significant global miRNA downregulation following exposure to hypoxia ( Fig. 2a and Supplementary data 1 ). Analysis of precursor and mature miRNA levels from deep-sequencing data revealed significant downregulation of mature miRNAs, compared with their precursors ( Fig. 2b and Supplementary data 2 ). Using quantitative reverse transcriptase–PCR, we analysed the expression of seven significantly downregulated miRNAs from Fig. 2a , in cells exposed to normoxia or hypoxia. There was a significant increase in pri-miRNA levels of six of seven miRNAs that were tested ( Fig. 2c ). There was also significant downregulation of corresponding mature miRNA levels in response to hypoxia ( Fig. 2d ), suggesting defective processing machinery under hypoxia conditions. These data were further validated by northern blot analysis of miR-16a and 27a in cancer cells exposed to normoxia and hypoxia ( Supplementary Fig. 4a ). 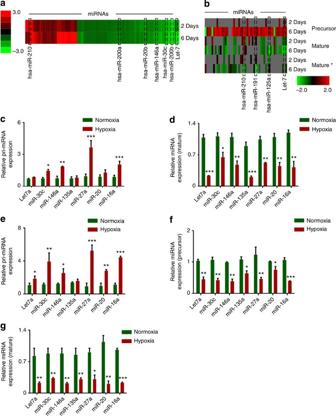Figure 2: Hypoxia-mediated downregulation in Drosha and Dicer results in decreased miRNA levels. (a) Heat map showing mature miRNA levels under hypoxic conditions, assessed using miRNA array data. (b) Heat map showing precursor miRNA levels under hypoxic conditions, along with the corresponding mature sense (mature) and antisense (mature*) levels. (c,d) Pri-miRNA and mature miRNA expression levels of significantly altered miRNAs under hypoxia exposure in A2780 cells. (e) Pri-miRNA levels in RNA extracted from nuclear fractionated A2780 cells treated with normoxia and hypoxia. (f,g) Precursor and mature miRNA levels in RNA extracted from cytoplasmic fraction of A2780 cells treated with normoxia and hypoxia. Data are presented as mean±s.e.m. ofn≥3 experimental groups. *P<0.05, **P<0.01, ***P<0.001 (Studentt-test). Figure 2: Hypoxia-mediated downregulation in Drosha and Dicer results in decreased miRNA levels. ( a ) Heat map showing mature miRNA levels under hypoxic conditions, assessed using miRNA array data. ( b ) Heat map showing precursor miRNA levels under hypoxic conditions, along with the corresponding mature sense (mature) and antisense (mature*) levels. ( c , d ) Pri-miRNA and mature miRNA expression levels of significantly altered miRNAs under hypoxia exposure in A2780 cells. ( e ) Pri-miRNA levels in RNA extracted from nuclear fractionated A2780 cells treated with normoxia and hypoxia. ( f , g ) Precursor and mature miRNA levels in RNA extracted from cytoplasmic fraction of A2780 cells treated with normoxia and hypoxia. Data are presented as mean±s.e.m. of n ≥3 experimental groups. * P <0.05, ** P <0.01, *** P <0.001 (Student t -test). Full size image Next, to understand the individual contribution of Drosha and Dicer downregulation in the miRNA processing downregulation, we carried out quantification of pri, precursor and mature miRNAs in RNA from nuclear and cytoplasmic fractionated A2780 cells exposed to normoxia or hypoxia. RNA from nuclear fractionated samples had significantly upregulated pri-miRNA levels ( Fig. 2e ), consistent with the total RNA data in Fig. 2c . Interestingly, we noted >40% reduction in precursor miRNA levels in hypoxia-treated samples compared with normoxia ( Fig. 2f ). In addition, samples from hypoxia-exposed cells had >60% reduction in mature miRNA levels compared with normoxia in the cytoplasmic fraction ( Fig. 2g ). Using the ovarian cancer data from the Cancer Genome Atlas project (TCGA), we investigated the effect of low Drosha and Dicer levels on mature miRNA levels and observed that most miRNAs (>80%) were affected by downregulation of Drosha and Dicer ( Supplementary Fig. 4b ). In the TCGA data set, we observed significantly worse median overall survival with low Drosha and Dicer levels ( Supplementary Fig. 4c ). Using a hypoxia metagene signature [22] , we examined the survival difference between patients with high versus low hypoxia levels in their tumours, according to the TCGA data. We observed significantly worse survival rates in patients whose tumours had high levels of hypoxia ( Supplementary Fig. 4d ). Drosha is downregulated by ETS family members Next, we investigated the mechanism by which hypoxia could regulate Drosha expression. There was no significant change in Drosha mRNA half-life under hypoxic conditions ( Supplementary Fig. 5a ), pointing to transcriptional regulation of Drosha. Interestingly, we observed a small change in Dicer mRNA half-life under hypoxia ( Supplementary Fig. 5b ). Luciferase activity for the Drosha and Dicer promoters showed a significant decrease in Drosha promoter luciferase activity after exposure to hypoxia in A2780 cancer cells ( Fig. 3a and Supplementary Fig. 5c ). In addition, there was no significant change in Drosha protein half-life with hypoxia, suggesting that the mechanism is likely to be transcriptional ( Supplementary Fig. 5d ). 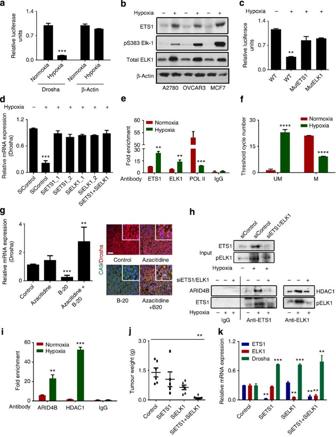Figure 3: Drosha is downregulated by the ETS1/ELK1 complex under hypoxic conditions. (a) Relative luciferase reporter activity for the Drosha promoter region under hypoxic conditions. β-Actin was used as a control. (b) Protein expression of ETS1 and ELK1 under hypoxic conditions in various cell lines. (c) Luciferase reporter activity for the wild-type (WT) Drosha promoter region and the ETS1 or ELK1 binding site–mutant Drosha promoter region under hypoxic conditions. (d) Drosha mRNA expression levels after ETS1, ElK1 and ETS/ELK1 siRNA gene knockdown under hypoxic conditions. (e) Anti-ETS1, anti-ELK1 and anti-POL II chromatin immunoprecipitation assay results showing fold enrichment of ETS1, ELK1 and POL II binding to the Drosha promoter region in A2780 cells. Rabbit IgG was used as a control and real-time PCR was used to quantitate the fold enrichment. (f) Effect of hypoxia on Drosha promoter methylation assessed by bisulfite conversion and methylation-specific PCR. The threshold cycle numbers obtained from samples with specific primers for unmethylated (UM) and methylated (M) sequences of the same promoter region of Drosha are shown. (g) mRNA and protein expression of Drosha in mouse tumour samples treated with B-20 (anti-VEGF antibody) and azacitidine. Scale bar, 200 μm. (h) Immunoprecipitation of hypoxia samples against ETS1 and ELK1 antibodies, probed for corresponding binding proteins ARID4B (ETS1) and HDAC1 (ELK1). (i) Anti-ARID4B and anti-HDAC1 chromatin immunoprecipitation assay results showing fold enrichment of ARID4B and HDAC1 binding to the Drosha promoter region in A2780 cells.(j) Aggregate tumour mass from tumours in the mouse orthotopic ovarian cancer model treated with control, ETS1, ELK1 and combination siRNAs. (k) Average mRNA expression of Drosha, ETS1 and ELK1 in the same tumour samples. All images shown are representative and data are presented as mean±s.e.m. ofn≥3 experimental groups. **P<0.01, ***P<0.001 (Studentt-test). Figure 3: Drosha is downregulated by the ETS1/ELK1 complex under hypoxic conditions. ( a ) Relative luciferase reporter activity for the Drosha promoter region under hypoxic conditions. β-Actin was used as a control. ( b ) Protein expression of ETS1 and ELK1 under hypoxic conditions in various cell lines. ( c ) Luciferase reporter activity for the wild-type (WT) Drosha promoter region and the ETS1 or ELK1 binding site–mutant Drosha promoter region under hypoxic conditions. ( d ) Drosha mRNA expression levels after ETS1, ElK1 and ETS/ELK1 siRNA gene knockdown under hypoxic conditions. ( e ) Anti-ETS1, anti-ELK1 and anti-POL II chromatin immunoprecipitation assay results showing fold enrichment of ETS1, ELK1 and POL II binding to the Drosha promoter region in A2780 cells. Rabbit IgG was used as a control and real-time PCR was used to quantitate the fold enrichment. ( f ) Effect of hypoxia on Drosha promoter methylation assessed by bisulfite conversion and methylation-specific PCR. The threshold cycle numbers obtained from samples with specific primers for unmethylated (UM) and methylated (M) sequences of the same promoter region of Drosha are shown. ( g ) mRNA and protein expression of Drosha in mouse tumour samples treated with B-20 (anti-VEGF antibody) and azacitidine. Scale bar, 200 μm. ( h ) Immunoprecipitation of hypoxia samples against ETS1 and ELK1 antibodies, probed for corresponding binding proteins ARID4B (ETS1) and HDAC1 (ELK1). ( i ) Anti-ARID4B and anti-HDAC1 chromatin immunoprecipitation assay results showing fold enrichment of ARID4B and HDAC1 binding to the Drosha promoter region in A2780 cells. ( j ) Aggregate tumour mass from tumours in the mouse orthotopic ovarian cancer model treated with control, ETS1, ELK1 and combination siRNAs. ( k ) Average mRNA expression of Drosha, ETS1 and ELK1 in the same tumour samples. All images shown are representative and data are presented as mean±s.e.m. of n ≥3 experimental groups. ** P <0.01, *** P <0.001 (Student t -test). Full size image To identify potential regulatory transcription factors, we carried out bioinformatics analyses using Matinspector and Matbase (Genomatix Inc.). In addition, we tested the role of previously reported transcription factors in the hypoxia-mediated downregulation of Drosha [23] , [24] , [25] . There was no significant change in Drosha following small interfering RNA (siRNA)-mediated silencing of Myc, nuclear factor-κB or SP-1 transcription factors ( Supplementary Fig. 5e ). From the bioinformatics analysis, ETS1 and ELK1 were found to have binding sites on opposite strands at very close proximity to the transcription initiation site ( Supplementary Fig. 5f ), and a previous study demonstrated transcriptional downregulation of downstream genes when ETS1/ELK1 bind to regions with very close proximity to the transcription initiation site [26] . Consistent with these findings, we observed an increase in both mRNA and protein levels of ETS1 and ELK1 under hypoxic conditions ( Fig. 3b and Supplementary Fig. 5g,h ). Of note, we also observed an increase in pELK1 levels, suggesting that ELK1 is activated under hypoxic conditions ( Fig. 3b ). In addition, we observed rescue of Drosha promoter activity in cells with mutations at the ETS1 or ELK1 binding sites under hypoxic conditions ( Fig. 3c and Supplementary Fig. 5i ). Previous studies have demonstrated HIF1α-dependent increase in ETS1 (ref. 27 ) and ELK1 via mitogen-activated protein kinase signalling [28] under hypoxia exposure. Nevertheless, we tested the potential role of loss of miRNA repression under hypoxia exposure, resulting in increased ETS1 and ELK1. In siDicer+siDrosha-treated cells, we did not observe any significant change in ETS1 or ELK1 expression ( Supplementary Fig. 6 ). Moreover, we tested for CA9 and VEGF changes in siDicer+siDrosha-treated cells and observed no significant changes in their expression ( Supplementary Fig. 6 ), ruling out the possibility that miRNA repression loss as a mechanism for CA9 or VEGF increase under hypoxia exposure. Next, we knocked down ETS1 and/or ELK1 to study the effect of these two proteins on Drosha levels ( Supplementary Fig. 7a,b ). Drosha expression was rescued after silencing ETS1, ELK1, or both, suggesting that ETS1 and ELK1 serve as transcriptional repressors for Drosha ( Fig. 3d and Supplementary Fig. 7c ). Chromatin immunoprecipitation assays with anti-ETS1 and anti-ELK1 were performed to confirm definitive binding of these elements in the promoter region. Compared with IgG or normoxic controls, significant enrichment in the binding of ETS1 and ELK1 to the promoter region of Drosha was observed in A2780 ( Fig. 3e and Supplementary Fig. 8a ) and MCF7 cells ( Supplementary Fig. 8b ) under hypoxic conditions. In addition, we observed a significant reduction in polymerase II occupancy at the Drosha promoter region under hypoxia conditions ( Fig. 3e ). To elucidate potential mechanisms by which ETS family members transcriptionally repress Drosha levels, we performed Ingenuity Pathway Network analysis. This analysis revealed that ETS1 could bind to the histone deacetylation-related molecule HDAC1, and that ELK1 could bind to the DNA methylation-related molecule ARID4B [29] , [30] ( Supplementary Fig. 9a ). A concentrated CpG island was observed near the Drosha promoter region where ETS1 and ELK1 bind ( Supplementary Fig. 9b ). Treatment of DNA samples with bisulphite and methylation-specific PCR analysis revealed a significant increase in methylation at the ETS1 and ELK1 binding regions ( Fig. 3f and Supplementary Fig. 9c ). Methylation-specific restriction enzyme (MSRE) treatment and PCR analysis showed significant methylation at the CpG islands at the Drosha promoter region following in vitro hypoxia exposure or in bevacizumab-treated in vivo tumour samples ( Supplementary Fig. 9d ). In addition, cells treated with siRNAs against ETS1 or ELK1 under hypoxia showed significant reversal of Drosha promoter methylation compared with cells treated with control siRNA ( Supplementary Fig. 9e ). Treatment of cells with the methylation inhibitor, azacitidine, or the HDAC1 inhibitor, valproic acid, under hypoxic conditions rescued Drosha levels, which was consistent with methylation-specific PCR or MSRE data ( Supplementary Fig. 10a ). In addition, in vivo tumour samples treated with azacitidine showed significant rescue of Drosha even under hypoxic conditions induced by anti-VEGF therapy (VEGF-targeted antibody, B-20), with a corresponding increase in ETS1 and ELK1 levels ( Fig. 3g and Supplementary Fig. 10b ). Cells treated with the HIF1α antagonist topotecan [31] under hypoxic conditions showed rescue of Drosha by suppressing ETS1 across several time points ( Supplementary Fig. 10c,d ), confirming the role of HIF1α-mediated signalling in ETS1 expression. Importantly, immunoprecipitation of ETS1 and ELK1 from hypoxia-treated cells showed clear binding of ARID4B and HDAC1, respectively; this binding was abrogated by treatment of cells with siETS1+siELK1 under hypoxia ( Fig. 3h and Supplementary Fig. 11 ). Next, we performed Drosha chromatin immunoprecipitation analysis using antibodies against ARID4B and HDAC1. There was a significant enrichment of ARID4B or HDAC1 binding in the Drosha promoter region under hypoxia exposure ( Fig. 3i ), confirming the role of ETS1-ARID4B and ELK1-HDAC1 complex in Drosha downregulation. In the A2780 mouse model of ovarian cancer, using DOPC (1,2-Dioleoyl-sn-glycero-3-phosphocholine) nanoliposomes to deliver siRNAs against ETS1, ELK1, or both, we observed significant tumour reduction in the tumours treated with siETS1 and siELK1; the lowest tumour weight was observed in the combination treatment group ( Fig. 3j ). Tumours from all three treatment groups showed increased expression of Drosha compared with the control group, and a significant reduction in ETS1 and ELK1 was observed in the treatment groups ( Fig. 3k ). In the MCF7 orthotopic breast cancer model, treatment with the combination of siETS1-DOPC and siELK1-DOPC resulted in similar biological effects, suggesting that ETS1- and ELK1-mediated Drosha deregulation is not limited to one particular cancer type ( Supplementary Fig. 12a–c ). To understand the clinical relevance to ETS1/ELK1 expression, we next examined the correlation of ETS1 and ELK1 with patient survival by analysing mRNA expression of ETS1 and ELK1 in human tumour samples ( n =75). Patients with high tumoral ETS1 or ELK1 expression had significantly lower survival compared with those with low ETS1 or ELK1 expression ( Supplementary Fig. 13a,b ). Functional effects of deregulated miRNA biogenesis To identify potential tumour-promoting pathways affected by hypoxia, we analysed mRNA expression data from deep sequencing coupled with miRNA expression data from miRNA array analysis of A2780 cells exposed to hypoxia and normoxia. Ingenuity Pathway Network analysis of mRNA and miRNA data from deep sequencing identified key novel miRNA–mRNA interactions that could potentially lead to enhanced tumour progression under hypoxic conditions ( Supplementary Data 3 and 4 ). MiR-200, a well-studied miRNA to play role in cancer growth and metastasis, was one among the hypoxia-activated networks identified ( Supplementary data 4 ). Pathway enrichment analyses revealed that cell adhesion, migration and growth networks were the most significantly upregulated pathways under hypoxic conditions ( Supplementary Fig. 14a ). Cells under hypoxic conditions had consistent upregulation of RHOB1, TAGLN, SERTAD1, TXNIP, JAG1, CTGF and JUN, while corresponding miRNAs let7a, miR-135a, miR-146a and miR-30c were significantly downregulated under hypoxic conditions ( Figs 4a,b and 2d,g ). Dicer and Drosha silencing under normoxia resulted in similar downregulation of the aforementioned miRNAs and corresponding upregulation of genes ( Fig. 4a,b ). Ectopic expression of Dicer and Drosha under hypoxia exposure resulted in rescue of the miRNAs and corresponding downregulation of mRNA targets ( Fig. 4a,b ). In addition, we tested the known miR-185 and HIF2α axis [15] in the A2780 cancer cells following exposure to hypoxia. MiR-185 was significantly downregulated along with corresponding upregulation of HIF2α ( Supplementary Fig. 14b ). In addition, rescue of miR-185 by Drosha and Dicer ectopic expression or delivery of miR-185 mimics under hypoxia exposure resulted in significant downregulation of HIF2α ( Supplementary Fig. 14b ). These data further support the role of hypoxia-mediated Dicer and Drosha deregulation in hypoxia signalling and tumour progression. 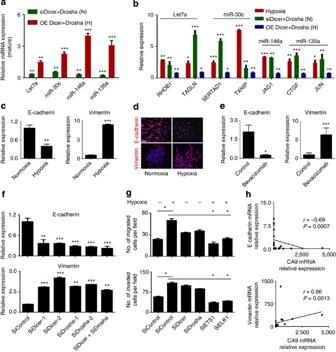Figure 4: Drosha and Dicer downregulation under hypoxia leads to increased epithelial-to-mesenchymal transition. Expression of significantly altered pro-miRNAs (a) and metastatic genes (b) in Dicer and Drosha knocked down A2780 cells under normoxia (data shown normalized to siControl) or ectopic expression of Dicer and Drosha under hypoxia (data shown normalized to control), N, normoxia; H, hypoxia. E-cadherin and vimentin mRNA (c) and protein (d) expression levels under hypoxic exposure in A2780 cells. Blue, nucleus. Scale bar, 200 μm. (e) mRNA levels of E-cadherin and vimentin in A2780 mouse tumour samples treated with bevacizumab. (f) E-cadherin (top) and vimentin (bottom) expression after knockdown of Dicer, Drosha, or both, using siRNAs in A2780 cells. (g) Effect of Drosha and Dicer on cell migration and invasion in A2780 cells. Drosha and Dicer levels were downregulated using siRNAs under normoxic conditions. Rescue of Drosha was achieved using siRNAs against ETS1 and ELK1 under hypoxic conditions. (h) Pearson correlation between E-cadherin or vimentin and hypoxia marker CA9 expression in clinical ovarian tumour samples (n=30). All images shown are representative and data are presented as mean±s.e.m. ofn≥3 experimental groups. *P<0.05, **P<0.01, ***P<0.001 (Studentt-test). Figure 4: Drosha and Dicer downregulation under hypoxia leads to increased epithelial-to-mesenchymal transition. Expression of significantly altered pro-miRNAs ( a ) and metastatic genes ( b ) in Dicer and Drosha knocked down A2780 cells under normoxia (data shown normalized to siControl) or ectopic expression of Dicer and Drosha under hypoxia (data shown normalized to control), N, normoxia; H, hypoxia. E-cadherin and vimentin mRNA ( c ) and protein ( d ) expression levels under hypoxic exposure in A2780 cells. Blue, nucleus. Scale bar, 200 μm. ( e ) mRNA levels of E-cadherin and vimentin in A2780 mouse tumour samples treated with bevacizumab. ( f ) E-cadherin (top) and vimentin (bottom) expression after knockdown of Dicer, Drosha, or both, using siRNAs in A2780 cells. ( g ) Effect of Drosha and Dicer on cell migration and invasion in A2780 cells. Drosha and Dicer levels were downregulated using siRNAs under normoxic conditions. Rescue of Drosha was achieved using siRNAs against ETS1 and ELK1 under hypoxic conditions. ( h ) Pearson correlation between E-cadherin or vimentin and hypoxia marker CA9 expression in clinical ovarian tumour samples ( n =30). All images shown are representative and data are presented as mean±s.e.m. of n ≥3 experimental groups. * P <0.05, ** P <0.01, *** P <0.001 (Student t -test). Full size image Consistent with the altered pathways described above, enhanced epithelial-to-mesenchymal transition (EMT) features were observed in cells under hypoxic conditions ( Supplementary Fig. 15a ). Analysis of EMT markers in various cell lines showed significantly decreased E-cadherin and increased vimentin mRNA and protein levels under hypoxic conditions ( Fig. 4c,d and Supplementary Fig. 15b,c ). RNA samples from the previously discussed bevacizumab-treated A2780 tumours showed reduced E-cadherin expression and increased vimentin expression, consistent with our in vitro observations ( Fig. 4e ). To elucidate the roles of Drosha and Dicer in the EMT process, we silenced Drosha and Dicer in A2780 and MCF7 cells, after which we observed significantly decreased E-cadherin and increased vimentin expression ( Fig. 4f and Supplementary Fig. 16a ). There was significant increase in migration and invasion of the A2780 or MCF7 cells after silencing of Dicer, Drosha, or both ( Fig. 4g and Supplementary Fig. 16b ). Correlative analysis of E-cadherin and CA9 in samples from patients with ovarian cancer showed a significant inverse correlation between E-cadherin and CA9 expression ( r =−0.69, P =0.0007). Vimentin expression, however, was positively correlated with CA9 expression ( r =−0.66, P =0.0013; Fig. 4h ). We created stable cell lines ectopically expressing Dicer and/or Drosha in HeyA8 ovarian cancer cells that have low basal Drosha/Dicer expression levels, and exposed the cells to hypoxia ( Supplementary Fig. 17a–c ). There was a significant reduction in EMT phenotype, including increased E-cadherin and decreased vimentin expression in HeyA8-control cells under hypoxia exposure. We observed disruption of hypoxia-mediated induction of EMT phenotype on rescue of Drosha and Dicer in these cells ( Supplementary Fig. 17d ). In addition, a reduction in migration and invasion was observed in all three cell line variants compared with control cells exposed to hypoxia ( Supplementary Fig. 17e,f ). Next, we ectopically expressed Drosha and Dicer in A2780 cells and tested their effects after hypoxia exposure ( Supplementary Fig. 17g ). There was significant reduction in the EMT phenotype in Drosha-, Dicer- or Drosha+Dicer-expressing cells compared with control cells exposed to hypoxia ( Supplementary Fig. 17g ). Next, to understand the biological roles that Drosha and Dicer play in tumour progression, we used an orthotopic model of ovarian cancer with luciferase-labelled A2780 cells implanted in the ovary. On knockdown of Drosha and Dicer using siRNAs (DOPC), we observed significant increases in aggregate tumour weight ( Fig. 5a ), and number and incidence of distant metastatic nodules ( Fig. 5b ) in the treatment groups compared with the control group. These findings are consistent with the increase in luciferase intensity observed in treatment groups ( Fig. 5c ). The tumour metastasis rate was significantly higher including rare sites such as the liver in the siDicer-DOPC, siDrosha-DOPC and combination treatment groups compared with the control group ( Fig. 5d and Supplementary Fig. 18a ), which showed metastatic lesions only in the mesentery. Reduction in Dicer or Drosha expression in respective treatment groups was also observed ( Fig. 5e ). Decreased E-cadherin and increased vimentin protein levels were observed in the siDicer, siDrosha and combination treatment groups compared with the control group ( Fig. 5f ). Similar increases in tumour weight and spread were observed with Drosha and Dicer knockdown in intraperitoneal ovarian cancer mouse models, resembling the clinical features of advanced-stage disease ( Supplementary Fig. 18b,c ). Treatment with siDicer+siDrosha also produced a similar pattern in the MCF7 mouse model of breast cancer with significant increases in tumour growth and metastatic rate being observed ( Supplementary Fig. 19a–d ). In the HeyA8 in vivo model of ovarian cancer, ectopically expression of Drosha, Dicer or Drosha+Dicer resulted in significant reduction in tumour weight ( Fig. 5g ) and number of distant metastatic nodules ( Fig. 5h ). 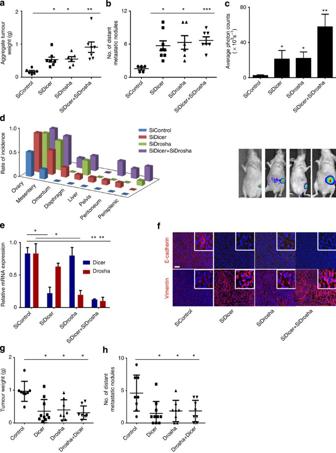Figure 5: Drosha and Dicer downregulation results in increased cancer progressionin vivo. Aggregate tumour weight (a) and number of distant metastatic nodules (b) in mice treated with siRNA against Dicer, Drosha, or both, compared with the control siRNA group (n=10 per group). (c) Average photon counts from each group of mice treated with siRNA against Dicer, Drosha, or both, compared with controls. Representative bioluminescence images are shown below the respective groups. (d) Distant metastatic nodule incidence rate in an orthotopic mouse model of ovarian cancer (left). (e) Drosha and Dicer mRNA expression in mouse tumour samples treated with siRNA against Dicer or Drosha. (f) Expression of epithelial-to-mesenchymal transition markers (E-cadherin, red; vimentin, red; nucleus, blue) in tumour samples from thein vivoexperiment groups. Scale bar, 200 μm. Aggregate tumour weight (g) and number of distant metastatic nodules (h) in mice implanted with HeyA8 cells ectopically expressing Dicer, Drosha and Dicer+Drosha. *P<0.05, **P<0.01, ***P<0.001 (Studentt-test). Figure 5: Drosha and Dicer downregulation results in increased cancer progression in vivo . Aggregate tumour weight ( a ) and number of distant metastatic nodules ( b ) in mice treated with siRNA against Dicer, Drosha, or both, compared with the control siRNA group ( n =10 per group). ( c ) Average photon counts from each group of mice treated with siRNA against Dicer, Drosha, or both, compared with controls. Representative bioluminescence images are shown below the respective groups. ( d ) Distant metastatic nodule incidence rate in an orthotopic mouse model of ovarian cancer (left). ( e ) Drosha and Dicer mRNA expression in mouse tumour samples treated with siRNA against Dicer or Drosha. ( f ) Expression of epithelial-to-mesenchymal transition markers (E-cadherin, red; vimentin, red; nucleus, blue) in tumour samples from the in vivo experiment groups. Scale bar, 200 μm. Aggregate tumour weight ( g ) and number of distant metastatic nodules ( h ) in mice implanted with HeyA8 cells ectopically expressing Dicer, Drosha and Dicer+Drosha. * P <0.05, ** P <0.01, *** P <0.001 (Student t -test). Full size image We next sought to determine whether treatment with siETS1/siELK1 could reverse the hypoxia-induced downregulation of miRNA biogenesis machinery following treatment with bevacizumab. Mice were treated with bevacizumab 2 weeks after tumour establishment. There was a significant increase in tumour weight and number of metastatic nodules in the bevacizumab treatment group ( Fig. 6a ). In mice treated with siETS1/siELK1, we observed significant reductions in tumour weight and number of metastatic nodules and spread compared with mice treated with bevacizumab alone ( Fig. 6b,c ). A significant increase in CA9 expression was observed in mice that received anti-VEGF therapy compared with control mice ( Fig. 6d ). Importantly, we noted rescue of Drosha expression in the siETS/ELK1 treatment group ( Fig. 6e ). Taken together, these data demonstrate the importance of Drosha in tumour progression as well as the role of ETS1/ELK1 in its regulation. 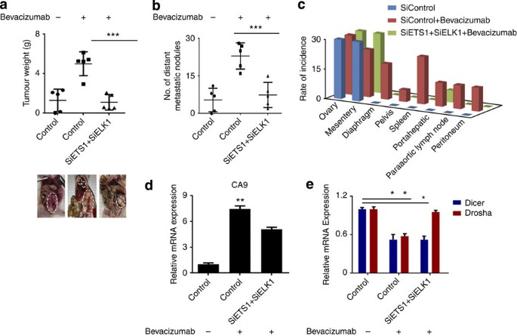Figure 6: Rescue of Drosha under anti-VEGF therapy results in decreased tumour progressionin vivo. (a,b) Effect of rescue of Drosha after anti-vascular endothelial growth factor (VEGF) therapy in A2780 model. Aggregate tumour weight is shown (a) and number of distant metastatic nodules (b) in mice treated with bevacizumab and mice treated with siRNAs against ETS+ELK1. Also shown are representative pictures of tumour burden (a, bottom) in all treatment groups (n=5 per group). (c) Distribution of metastatic nodules in individual mice groups treated with siDicer, siDrosha and siDicer+siDrosha. Hypoxia marker CA9 (d) and Dicer and Drosha (e) mRNA expression levels in the tumour samples from the mouse model. All images shown are representative and data are presented as s.e.m. ofn≥3 experimental groups. *P<0.05, **P<0.01, ***P<0.001 (Studentt-test). Figure 6: Rescue of Drosha under anti-VEGF therapy results in decreased tumour progression in vivo . ( a , b ) Effect of rescue of Drosha after anti-vascular endothelial growth factor (VEGF) therapy in A2780 model. Aggregate tumour weight is shown ( a ) and number of distant metastatic nodules ( b ) in mice treated with bevacizumab and mice treated with siRNAs against ETS+ELK1. Also shown are representative pictures of tumour burden ( a , bottom) in all treatment groups ( n =5 per group). ( c ) Distribution of metastatic nodules in individual mice groups treated with siDicer, siDrosha and siDicer+siDrosha. Hypoxia marker CA9 ( d ) and Dicer and Drosha ( e ) mRNA expression levels in the tumour samples from the mouse model. All images shown are representative and data are presented as s.e.m. of n ≥3 experimental groups. * P <0.05, ** P <0.01, *** P <0.001 (Student t -test). Full size image Our data show that tumour hypoxia plays a critical role in the downregulation of Drosha and Dicer, leading to downregulated miRNA biogenesis in cancer. Drosha is downregulated by ETS1 and ELK1 recruitment of HDAC1 and ARID4B onto the promoter region. ETS1/ELK1 silencing under hypoxic conditions in vivo rescued Drosha expression and led to significant reductions in tumour growth and metastasis ( Fig. 7 ). During progression, tumours encounter substantial hypoxia owing to abnormal vasculature [18] . Emerging studies have shown that hypoxia is involved in promoting tumour progression and resistance to therapy [18] , [19] . Direct assessment of tumour hypoxia in patient samples has demonstrated worse clinical outcomes in patients with high intratumoral hypoxia [20] . In addition, some studies suggest that anti-VEGF therapies induce substantial hypoxia in tumours [32] , [33] . Previous reports have shown hypoxia-mediated EMT via direct activation of Twist1 by HIF1α (ref. 34 ) or notch signalling [35] . Our findings provide a new understanding of the mechanisms by which hypoxia contributes to increased cancer metastasis via miRNA biogenesis downregulation. 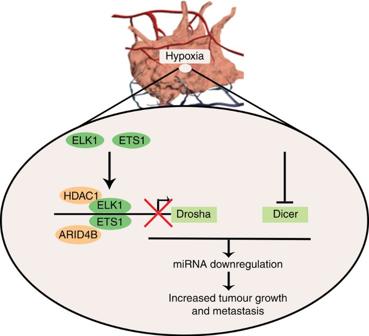Figure 7: Schematic representation. Schematic representation of mechanisms by which Drosha and Dicer downregulation in hypoxia results in increased cancer growth and metastasis. Figure 7: Schematic representation. Schematic representation of mechanisms by which Drosha and Dicer downregulation in hypoxia results in increased cancer growth and metastasis. Full size image Decreased expression of Drosha and Dicer in cancer is associated with poor clinical outcome [8] , [9] , [10] , [11] . Recent reports showed the association of Dicer with increased metastasis using a Dicer knockout [36] or a breast cancer model [37] . Our study provides further understanding of a previously unrecognized role of hypoxia in the regulation of Drosha and Dicer. Use of Drosha- and Dicer-independent siRNA-based gene targeting is an emerging strategy to develop therapies that target undrugable genes [38] , [39] , [40] . As suggested in this study, in vivo delivery of DOPC–siETS1/ELK1 nanoparticles serve as a promising approach to rescue expression of Drosha in cancer. Here we elucidated the mechanism by which Drosha is downregulated under hypoxia and provide new directions towards rescue of miRNA biogenesis in cancer. Moreover, a parallel study by van den Beucken et al. [17] describes a novel mechanism by which Dicer is downregulated under hypoxia. Altogether, a comprehensive understanding of Drosha and Dicer downregulation under hypoxic conditions is an important leap towards understanding the miRNA biogenesis defects that occur during cancer progression. Cell line maintenance and siRNA and miRNA transfections All cell lines were maintained in 5% CO 2 at 37 °C. Ovarian cancer (A2780, OVCAR3, SKOV3, OVCA432, HeyA8, IGROV, EG) and breast cancer (MDA-MB-231, MCF7, GILM2) cells were obtained from the American Type Culture Collection and were maintained in RPMI 1640 supplemented with 10–15% fetal bovine serum (FBS) and 0.1% gentamicin sulfate (GeminiBioproducts, Calabasas, CA). All cell lines were routinely tested to confirm the absence of Mycoplasma , and all in vitro experiments were conducted with 60–80% confluent cultures. All siRNA transfections ( Supplementary Table 1 ) were performed using RNAiMAX (Invitrogen, Carlsbad, CA) reagent using forward transfection protocol from the manufacturer. Media was changed 5 h after transfections to minimize toxicity. For all hypoxia treatments, cells were incubated in an oxygen-controlled hypoxia chamber at 1% O 2 . For ectopic expression of Drosha and Dicer, we obtained plasmids from Addgene (IDs 10828 and 25851, respectively). Next, we cloned open reading frames into pLKO.1-GFP or Puromycin lentiviral plasmids. We transduced HeyA8 cells with virus particles, and then selection using green fluorescent protein (Drosha) or puromycin (Dicer) was carried out to establish stable cell variants. In vivo models Female athymic nude mice were purchased from Taconic Farms (Hudson, NY). These animals were cared for according to guidelines set forth by the American Association for Accreditation of Laboratory Animal Care and the US Public Health Service policy on Human Care and Use of Laboratory Animals. All mouse studies were approved and supervised by The University of Texas MD Anderson Cancer Center Institutional Animal Care and Use Committee. All animals used were 8–12 weeks old at the time of injection. Orthotopic models of ovarian cancer were developed as described previously [41] , [42] . For all animal experiments, cells were harvested using trypsin-EDTA, neutralized with FBS-containing media, washed and resuspended to the appropriate cell number in Hanks’ balanced salt solution (HBSS; Gibco, Carlsbad, CA) before injection. For the A2780 model, cells were injected either intraperitoneally (1 × 10 6 cells in 200 μl of HBSS) or directly into the ovary (0.8 × 10 6 cells in a 1:1 mixture of BD Matrigel and HBSS with a total volume of 100 μl of HBSS). For the HeyA8 cells and variants expressing Drosha, Dicer and Drosha+Dicer (0.8 × 10 6 cells in a 1:1 mixture of BD Matrigel and HBSS with a total volume of 100 μl of HBSS), intra-ovarian injections were performed. For the breast cancer model, MCF7 cells were injected into the mammary fat pad (5 × 10 6 cells in a 1:1 mixture of BD Matrigel and HBSS). For the intra-ovary injections, mice were anaesthetized with ketamine and xylazine. An incision just above the approximate site of the right ovary was made to visualize the ovary. A 1-ml tuberculin syringe with a 30-gauge needle was used to inject the cell suspension directly into the ovary. After injection, the incision was closed using surgical clips and the mouse was returned to a cage until fully recovered. For the orthotopic breast cancer model, the MCF7 cell mixture was injected into the second mammary fat pad from the top after the mouse was anaesthetized with ketamine and xylazine. One week before the injection of breast cancer cells, a 60-day release pellet containing 0.72 mg of 17β-estradiol (Innovative Research of America, Toledo, OH) was implanted subcutaneously into each mouse. For all therapeutic experiments, a dose of 200 μg siRNA/kg was used, as described previously [39] , [42] , [43] . For all models, unless indicated otherwise, twice weekly treatments were started 1 week after cell injection and continued for approximately 4 weeks. For miRNA or siRNA experiments, mice were randomly divided and treated with siRNA incorporated in neutral DOPC nanoliposomes (intraperitoneal administration). For the anti-VEGF therapy experiment, mice were allowed to develop tumours for 2–3 weeks and then two treatments of bevacizumab (6.25 mg kg −1 ) were administered. For the Drosha and Dicer rescue experiment, treatment with bevacizumab started on day 7 after cell implantation and continued until the end of the experiment. In all experiments, once mice in any group became moribund they were killed and necropsied, and tumours were harvested. Tumour weight and number and location of tumour nodules were recorded. Tumour tissue was either fixed in formalin for paraffin embedded, frozen in optimal cutting temperature media to prepare frozen slides, or snap-frozen for lysate preparation. Tumour samples Tumour samples were obtained after the study was approved [8] by the Institutional Review Board, and written informed consent was obtained from the patients for the use of clinical specimens for research. We obtained 75 specimens of invasive epithelial ovarian cancer from the MD Anderson Cancer Center Tumor Bank. For use as control samples, 15 normal ovarian epithelial samples were also obtained. Frozen tumour samples (~0.2 mg each) were used for total RNA isolation using Trizol method. TCGA data and bioinformatics analysis Bioinformatics analysis was performed in R (version 2.14.2; http://www.r-project.org ). Statistical significance was set at P <0.05. We downloaded and analysed publicly available data from the TCGA ( http://tcga-data.nci.nih.gov/ ) for patients with high-grade serous ovarian carcinoma. Level 3 Illumina RNASeq and miRNASeq were used to measure mRNA and miRNA expression. miRNASeq data were derived from the ‘isoform_quantification’ files from the ‘reads per million miRNA mapped’ values for mature forms of each microRNA. A list of 99 genes that comprised the hypoxia metagene was obtained from Winter et al. [22] Univariate Cox analysis was performed and ten genes with hazard ratio >1.1 ( KCTD11 , TNS4 , TUBB2A , ANGPTL4 , TEAD4 , DPM2 , PYGL , TPI1 , C16orf74 and ADORA2B ) were selected for further study. The median of the distribution was calculated for each patient. For survival analysis, the patients were grouped into percentiles according to the hypoxia metagene signature described above. We checked for an association between hypoxia signature and overall survival by choosing a cutoff to optimally split the samples into two groups and the log-rank test was employed to determine the significance of the association. To examine the association between Drosha and Dicer levels and overall survival, the patients were grouped into sextiles according to DICER and DROSHA expression. We compared all groups and obtained the best separation (minimal log-rank test P -value) for the groups linked to a positive association: DICER expression last sextile and DROSHA expression last sextile with DICER expression first sextile and DROSHA expression first sextile. We also compared miRNA levels between two additional groups: good responders and bad responders. Liposomal nanoparticle preparation miRNA or siRNA for in vivo intratumour delivery was incorporated into DOPC, as previously described [43] . DOPC and siRNA were mixed in the presence of excess tertiary butanol at a ratio of 1:10 (w/w) siRNA:DOPC. Tween 20 was added to the mixture in a ratio of 1:19 Tween 20:siRNA/DOPC. The mixture was vortexed, frozen in an acetone/dry ice bath and lyophilized. Before in vivo administration, this preparation was hydrated with PBS at room temperature at a concentration of 200 μg siRNA per kg per injection. miRNA microarray and deep sequencing Total RNA was extracted from the A2780 cells under normoxic or hypoxic conditions using the mirVana RNA Isolation kit (Ambion). RNA purity was assessed using Nanodrop spectrophotometric measurement (Thermo Scientific, Pittsburgh, PA) of the OD260/280 ratio with acceptable values falling between 1.9 and 2.1, as well as using Agilent Bioanalyser (Agilent Technologies, La Jolla, CA) with a RNA Integrity Number (RIN) number of at least 8. Five hundred nanograms of total RNA was used for labelling and hybridization, according to the manufacturer’s protocols (Agilent Technologies). Expression levels of miRNAs in ovarian cancer cells on exposure to hypoxia (1% O 2 ) were profiled using miRNA microarray (Agilent v14). Bioinformatic analysis was performed in R (version 2.14.2). Statistical significance was set at P <0.05. The raw intensity for each probe was the median feature pixel intensity with the median background subtracted, and setting an offset 1 ensured that no negative values would appear after log-transforming the data. Data were quantile-normalized and log2 transformed. A two-sided t -test was applied to determine significantly different miRNAs between samples. Heat maps were generated using the heat plot function of the library. Starting with 3 μg of total RNA for each sample, ribosomal RNA was depleted using Ribominus (Invitrogen/Life Technologies, Inc., Carlsbad, CA), following the manufacturer’s recommendations. Sequencing libraries were then prepared and barcoded individually using the SOLiD Total RNA-Seq Kit for Whole Transcriptome Libraries (Life Technologies), following the manufacturer’s recommendations. Prepared samples were then pooled and sequenced using the Life Technology 5500xl sequencer using 75 base forward read only. Data were extracted from XSQ files containing the read sequences, quality values were loaded onto a compute cluster and the reads were mapped in colorspace using the Life Technologies LifeScope 2.5.1 software, using default parameters. Reads were mapped to the human genome (hg19) downloaded from the UCSC Genome Bioinformatics Site ( http://genome.ucsc.edu ). The hg19 genome was slightly modified by deleting the Y chromosome to make a female genome. An hg19 exon reference file provided by Life Technologies was required by LifeScope to create the exon junction libraries needed to map reads that cross exon boundaries. This file was derived from the refGene database from UCSC. A human filter reference file was required (provided by Life Technologies) that contains the sequences of ribosomal and repetitive regions of the genome to filter reads that mapped to those regions. Mapped reads were output in the standard BAM (Binary Alignment/Map) format. BAM files were imported into Partek Genomics Suite 6.6 (Partek Incorporated, St Louis, MO) for gene expression analysis. Mapped reads contained in the BAM files were cross-referenced against the RefSeq database (downloaded from UCSC Genome Browser) and a small RNA database (UCSC Genome Browser) to generate RPKM (reads per kilobase of exon per million mapped reads) values for each gene. Low-expressing genes were excluded. Differential expression using the derived RPKM values was performed using analysis of variance. Genes with a false discovery rate <5% were considered significant. Significantly deregulated miRNAs from the miRNA array and mRNA data from deep sequencing were uploaded onto Ingenuity Pathway Network analysis (Ingenuity Systems, www.ingenuity.com ) and a network analysis with miRNA–mRNA target analysis was carried out to identify potential gene deregulation as a result of miRNA changes under hypoxic conditions. Immunoblotting Lysates from cultured cells were prepared using modified RIPA buffer (50 mM Tris–HCl (pH 7.4), 150 mM NaCl, 1% Triton, 0.5% deoxycholate) plus 25 μg ml −1 leupeptin, 10 μg ml −1 aprotinin, 2 mM EDTA and 1 mM sodium orthovandate. The protein concentrations were determined using a BCA Protein Assay Reagent kit (Pierce Biotechnology, Rockford, IL). Lysates were loaded and separated on SDS–PAGE. Proteins were transferred to a nitrocellulose membrane by semidry electrophoresis (Bio-Rad Laboratories, Hercules, CA) overnight, blocked with 5% BSA for 1 h and then incubated at 4 °C overnight with primary antibody (Dicer 1:1,000, Drosha 1:1,000 (Novus Biologicals, Littleton, CO), ETS1 1:500, ELK1 1:1,000, pELK1 1:500 (Cell signaling, Danvers, MA)). After washing with tris-buffered saline with Tween 20, the membranes were incubated with horseradish peroxidase-conjugated horse anti-Mouse or Rabbit IgG (1:2,000, GE Healthcare, UK) for 2 h. Horseradish peroxidase was visualized using an enhanced chemiluminescence detection kit (Pierce Biotechnology). To confirm equal sample loading, the blots were probed with an antibody specific for β-actin (0.1 μg ml −1 ; Sigma). Immunoprecipitation using antibodies against ETS1 or ELK1 was carried out using the Universal Magnetic Co-IP Kit (Active Motif, Carlsbad, CA), according to instructions provided by the company. Samples were processed for western blotting as described above. Using the antibody against ARID4B (Novus Biologicals) and HDAC1 (Cell Signaling), pull-down samples were probed for interactions. Full blottings are shown in Supplementary Figs 20 and 21 . Quantitative real-time PCR For mRNA quantification, total RNA was isolated using the Qiagen RNeasy kit (Qiagen, CA). Using 1,000 ng of RNA, complementary DNA was synthesized using a Verso cDNA kit (Thermo Scientific, PA), as per the manufacturer’s instructions. Analysis of mRNA levels was performed on a 7500 Fast Real-Time PCR System (Applied Biosystems, CA) with SYBR Green-based real-time PCR for all genes, except the one specified. Dicer and Drosha Taqman assays (Life Technologies) were performed. Specific primers used are described in Supplementary Table 1 . Semi-quantitative real-time PCR was done with reverse-transcribed RNA and 100 ng μl −1 sense and antisense primers in a total volume of 20 μl. For miRNA quantification, total RNA was isolated using Trizol (Invitrogen) extraction. RNA was isolated from nuclear and cytoplasmic fractionated cells using Paris kit (Life Technologies). Fractionation purity was confirmed by running the samples on agarose gel electrophoresis and visualization of precursor rRNA bands, 18 s, and 28 s rRNA bands. For pri-miRNA and mature miRNA quantifications, taqMan miRNA assays (Life Technologies) were used and reverse transcription, real-time PCR were carried out, according to the manufacturer’s instructions. Precursor miRNAs were quantified using c miRscript precursor miRNA assays (Qiagen). RNU6B (for mature miRNAs) or 18S (pri and precursor miRNAs) were used as a housekeeping gene. Immunostaining Staining was performed on optimal cutting temperature-embedded frozen tissue sections. Protein blocking of nonspecific epitopes was performed using 4% fish gelatin in tris-buffered saline with Tween 20 for 20 min. Slides were incubated with the primary antibody for Dicer, Drosha (Novus Biologicals, CA), E-cadherin (BD Transduction Laboratories, CA) or vimentin (Cell Signaling, CA) overnight at 4 °C. For immunofluorescence, secondary antibody staining was performed using either Alexa 594 or Alexa 488 (Molecular Probes). Nuclear staining was performed using Hoechst 33342 (Molecular Probes). Immunofluorescent images were captured using a Zeiss Axioplan 2 microscope and Hamamatsu ORCA-ER digital camera (Carl Zeiss Inc., Germany) Bright-field light images of haematoxylin and eosin-stained lung tissue sections were obtained using a Nikon Microphot-FXA microscope and Leica DFC320 digital camera (Nikon, Japan; Leica, Germany). From each group, ten images were taken at random and analysed for micrometastases, as well as scored for percentage of micrometastatic nodules. Migration and invasion assays Modified Boyden chambers (Coster, MA) coated with 0.1% gelatin (migration) or extracellular matrix components [44] (invasion) were used. A2780 or MCF7 cells (1 × 10 5 ) suspended in 100 μl of serum-free media were added into the upper chamber 24 h after siRNA transfections. Complete media for cells containing 10% FBS (500 μl) was added to the bottom chamber as a chemo-attractant. The chambers were incubated at 37 °C in 5% CO 2 for 6 h (migration) or overnight (invasion). After incubation, the cells in the upper chamber were removed with cotton swabs. Cells were fixed and stained, and counted using light microscopy. Cells from five random fields were counted. Experiments were done in duplicate and performed three times. MSP and MSRE analysis For MSP, MethPrimer ( http://www.urogene.org/methprimer/ ) software was used for the prediction of the CpG island of the Drosha promoter region and for design of methylation-specific primers ( Supplementary Table 1 ). Total DNA was isolated from normoxia- and hypoxia-treated cells using Phenol:Chloroform extraction and then treated with bisulfite using a methylation kit (EZ DNA Methylation-Gold; Zymo Research, CA). Using real-time PCR, as described above, quantification of methylation in hypoxia samples was performed by comparing them with normoxia samples. For MSRE analysis, primers were designed flanking the CpG island predicted by MethPrimer with at least two CpG islands on primers as suggested by qMethyl Light (Zymo Research). DNA samples from hypoxia- and normoxia-exposed cancer cells were subjected to MSREs provided in the kit. Following MSRE digestion of DNA, quantification of methylation was carried out using real-time PCR. Percentage methylation was calculated by comparing Ct values obtained from test (with MSRE) and reference (no MSRE) reactions as outlined in the kit manual. Northern blot analysis RNA from cells treated with normoxia and hypoxia were subjected to northern blot analysis using non-radioactive biotin-probe method [45] . Briefly, total RNA from A2780 cells exposed to normoxia and hypoxia was loaded onto 15% urea gel, electrophoresed and transferred to nylon membranes at 10–15 V (90 min) using Trans-Blot SD Semi-Dry Transfer Cell (Bio-Rad, CA). RNA was cross-linked to the membrane using ultraviolet cross-linker. For miRNA and U6 probes, pre-synthesized locked nucleic acid (LNA)-modified oligonucleotides were purchased from Exiqon ( http://www.exiqon.com ) with biotin conjugation. Hybridization and washing of the membranes were carried out using Northern max kit (Life Technologies) according to the manufacturer’s recommended protocol. Membranes were developed using Chemiluminescent Nucleic Acid Detection Module (Pierce Biotechnology). Actinomycin D mRNA stability assay Drosha or Dicer mRNA stability under hypoxic and normoxic conditions was assessed using 5 μg ml −1 (ref. 46 ) actinomycin D. Cells were grown in hypoxic or normoxic conditions for various time periods with or without actinomycin D. At specified time points, RNA was isolated and RNA levels of Drosha and Dicer were measured using real-time PCR, as described above. 18S was used to normalize between the hypoxia and normoxia samples. To assess RNA decay rates, Drosha and Dicer levels under hypoxic conditions after normalization with 18S were compared with Drosha and Dicer levels under normoxic conditions. Chromatin hybridization and immunoprecipitation assay Cells were cultured in hypoxic or normoxic conditions for 48 h and chromatin immunoprecipitation assays were performed using the Chip-it express kit (Active Motif), as described by the manufacturer. In brief, cross-linked cells were collected, lysed, sonicated and subjected to immunoprecipitation with the ETS1, ELK1, ARID4B and HDAC1 antibodies or IgG isotype control. Immunocomplexes were collected with protein A/G agarose magnetic beads and eluted. Cross-links were reversed by incubating at 65 °C with high salt concentration. PCR-based quantification of fold enrichment in ETS1 or ELK1 binding on the Drosha promoter region (primers used are in Supplementary Table 1 ) was performed. The 2,500–3,000 base upstream region of the ETS1 or ELK1 binding region was used as a control. Microdissection and RNA isolation In vivo tumour samples from a previous study [47] injected with Hypoxyprobe (Hypoxyprobe Inc., Burlington, MA) were used for the present study. Frozen sections (10 μm) were affixed onto polyethylene terephthalate slides (Leica), fixed in cold acetone (10 min), washed in PBS three times, stained for Hypoxyprobe using fluorescein isithiocyanate-conjugated antibody for 1 h on top of ice, washed and air-dried, and immediately followed by dissection. Microdissection was performed using an MD LMD laser microdissecting microscope (Leica). RNA was isolated from same samples using the Cells to Ct Kit (Applied Biosystems), according to manufacturer instructions. Real-time PCR was carried out to quantify gene expression. Transcription factor binding analysis and luciferase assays The promoter region of Drosha was analysed for potential transcription factor binding using Matinspector (Genomatix Inc., Germany), followed by analysis for a potential gene suppression role using LitInspector (Genomatix). The Drosha promoter luciferase reporter assay was performed in A2780 and MCF7 cells using the Dual Luciferase system (SwitchGear Genomics). Cells were transfected using FuGENE HD TFX reagent in a 96-well plate with empty promoter or Drosha promoter (Switchgear Genomics), along with the Cypridina TK control construct (pTK-Cluc). Cells were treated with hypoxia or normoxia for 48 h and luciferase activity was measured using the kit as described above. Mutation in the ETS1 or ELK1 binding region in the Drosha promoter was created using the Quick change site-directed mutagenesis kit (Agilent Technologies) and verified by sequencing. Primers used for mutagenesis are listed in Supplementary Table 1 . Accession codes: GEO accession number for micro array and RNA sequencing data: GSE5274 . How to cite this article: Rupaimoole, R. et al. Hypoxia-mediated downregulation of miRNA biogenesis promotes tumour progression. Nat. Commun. 5:5202 doi: 10.1038/ncomms6202 (2014).